Cross-species identification of genomic drivers of squamous cell carcinoma development across preneoplastic intermediates Cutaneous squamous cell carcinoma (cuSCC) comprises 15–20% of all skin cancers, accounting for over 700,000 cases in USA annually. Most cuSCC arise in association with a distinct precancerous lesion, the actinic keratosis (AK). To identify potential targets for molecularly targeted chemoprevention, here we perform integrated cross-species genomic analysis of cuSCC development through the preneoplastic AK stage using matched human samples and a solar ultraviolet radiation-driven Hairless mouse model. We identify the major transcriptional drivers of this progression sequence, showing that the key genomic changes in cuSCC development occur in the normal skin to AK transition. Our data validate the use of this ultraviolet radiation-driven mouse cuSCC model for cross-species analysis and demonstrate that cuSCC bears deep molecular similarities to multiple carcinogen-driven SCCs from diverse sites, suggesting that cuSCC may serve as an effective, accessible model for multiple SCC types and that common treatment and prevention strategies may be feasible. Actinic keratoses (AK) are likely the most common precancerous lesion in humans, affecting up to 5.5% of women and 13.9% of men in USA, accounting for 5.2 million outpatient visits per year at an estimated annual cost of over $1 billion [1] , [2] . AKs are scaly lesions, often readily appreciated on sun-exposed skin. Histologically, they are characterized by epidermal dysmaturation and partial thickness basal and spinous layer atypia. In time, this atypia may extend to the full thickness of the epidermis (AK3/squamous cell carcinoma in-situ) or beyond, culminating in invasive cutaneous squamous cell carcinoma (cuSCC). Ultraviolet radiation (UVR) is the main aetiological factor implicated in AK and cuSCC pathogenesis. Approximately 0.6% of clinically diagnosed AKs are estimated to progress to cuSCC within 1 year and 2.6% are estimated to progress within 4 years [3] . Thus, the standard practice of destroying these lesions is well founded, but there is still no rationally designed way of preventing their progression, and there are still up to 700,000 cases of cuSCC in USA every year [4] . Destructive therapies are effective but management of high-risk populations such as organ transplant recipients is challenging and systemic compounds such as retinoids have substantial adverse reactions [2] , [5] . AKs are almost always treated, usually quickly and easily on an outpatient basis; however, the morbidity and economic burden of multiple treatments is high [2] , [5] . Understanding the genetic alterations that dictate AK formation and progression to cuSCC forms the molecular basis for rationally designed targeted cancer chemoprevention for an extremely common skin cancer. To date, molecular genetic studies of AK have largely centred on known tumour suppressor genes. TP53 , RAS , CDKN2A mutations and loss of CDKN2A and p53 expression have been identified in AK [6] , [7] , [8] , as well as extensive loss-of-heterozygosity and chromosomal aberrations [9] . What dictates whether or not AKs progress to cSCC is inadequately understood as these genetic lesions are also commonly found in cuSCC. Amplifications of epidermal growth factor receptor ( EGFR ) and c-MYC have been identified in AK and cuSCC [10] , [11] . Loss of INPP5A and CKS1B amplification have been demonstrated in human cuSCC and smaller proportions of AKs [12] , [13] . Gene signatures that distinguish SCC from AK or irradiated skin have been identified, but they have not been refined to identify a mechanistic basis for progression [14] , [15] , [16] . Few of the multiple attempts at genome-wide analysis of AK and cuSCC [15] , [17] , [18] , [19] , [20] , [21] have used matched histologically validated lesions from individual patients [16] and all have employed several platforms known to have potentially high annotation error rates [22] . Given these challenges, it is not surprising that it has been difficult to identify drivers of progression when comparing tumour tissue to their normal counterparts, or when comparing unmatched samples. In this study, we sought to identify important genetic events that drive squamous cell carcinoma (SCC) development through combined analysis of next-generation sequencing of matched patient samples with a UVR-driven mouse model to identify key pathways. Our approach minimizes the impact of inter-individual variability and annotation errors, while enabling identification of the most biologically significant pathways through cross-species analysis. We compared non-lesional, chronically UVR-exposed skin (normal skin, ‘NS’ in human, ‘CHR’ in mouse) to preneoplastic AK (human)/papilloma (mouse) and subsequently to cuSCC using successive pairwise comparisons as well as progression models to highlight potential targets for cancer prevention. 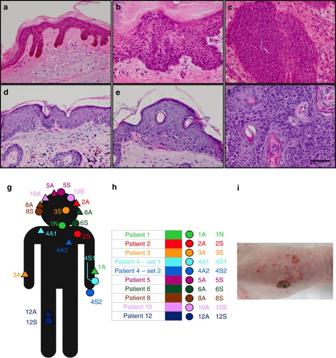Figure 1: Anatomic distribution and histology of representative tissues isolated from human patients and Hairless mice. (a–c) Normal (peri-tumoural) skin, actinic keratosis and invasive cuSCC, respectively, are shown from human patients. Scale bar, 50 μm. Human samples were processed following combined RNAlater and formalin fixation, resulting in significant cytoplasmic shrinkage. (d–f) Normal (peri-tumoural) skin, papillomas and invasive cuSCC, respectively, are shown from Hairless mice. (g) Anatomic locations of matched samples from human patients. (h) Tabular list of matched samples from human patients: (S) denotes the cuSCC with adjacent NS, (N) denotes normal skin and (A) denotes the AK. For patient 1, only NS and AK were available for analysis. (i) Representative skin samples from Hairless mice are shown, which include smaller papillomas and a smaller number of invasive carcinomas. Patient samples and mouse model A total of 27 tissue samples were isolated from nine patients who were treated for invasive cuSCC with Mohs surgery ( Table 1 ). cuSCC tumour cores were extracted before Mohs surgery with matched samples of peri-tumoural clinically normal skin within 1 cm of the tumour removed in the course of reconstruction. For most patients, a distinct AK was also isolated, often from the same general field ( Fig. 1a–c,g,h ). Table 1 Clinico-pathological characteristics of patient cohort and sequencing performed. Full size table Figure 1: Anatomic distribution and histology of representative tissues isolated from human patients and Hairless mice. ( a – c ) Normal (peri-tumoural) skin, actinic keratosis and invasive cuSCC, respectively, are shown from human patients. Scale bar, 50 μm. Human samples were processed following combined RNAlater and formalin fixation, resulting in significant cytoplasmic shrinkage. ( d – f ) Normal (peri-tumoural) skin, papillomas and invasive cuSCC, respectively, are shown from Hairless mice. ( g ) Anatomic locations of matched samples from human patients. ( h ) Tabular list of matched samples from human patients: (S) denotes the cuSCC with adjacent NS, (N) denotes normal skin and (A) denotes the AK. For patient 1, only NS and AK were available for analysis. ( i ) Representative skin samples from Hairless mice are shown, which include smaller papillomas and a smaller number of invasive carcinomas. Full size image In parallel, we established chronically UVR-irradiated SKH-1E Hairless mice using solar simulators (Oriel) as a highly relevant model for UVR-induced human cuSCC [23] , [24] ( Fig. 1d–f,i ). SKH-1E hairless mice are highly susceptible to UVR-induced skin tumours, UVR-induced immunosuppression and DNA damage [23] . Solar simulators more accurately simulate terrestrial UVR exposure than do fluorescent ultraviolet bulbs [24] . Thus our model ensures a useful platform in which we can test chemoprevention approaches. Tumours in these mice develop p53 (ref. 25 ), RAS (ref. 26 ) and CDKN2A (ref. 27 ) mutations in similar proportions to those in human cuSCC, along with copy number variations that map to ones reported in human cuSCC (chromosomes 3p, 11p and 9q) (refs 28 , 29 , 30 ) Serial Analysis of Gene Expression (SAGE) mRNA gene expression data from this model, comparing UVR-induced cuSCC to NS epidermis, shows substantially similar patterns of changes to our human data including overexpression of matrix metalloproteinases and hyperproliferative keratins [31] . Importantly, these mice develop precancerous papillomas (PAP) and cuSCC following chronic low-dose UVR exposure [23] . Six littermate female Hairless mice were chronically irradiated with 12.5 kJ m −2 of ultraviolet B (UVB) weekly for 100 days, and 14 days following cessation of irradiation, killed at which time, chronically irradiated skin (CHR), PAP, and cuSCC were isolated. All papillomas were grade 1 or grade 2 (not grade 3) and all cuSCC were grade 1 or grade 2 (ref. 23 ). All human and mouse samples were histologically validated with estimated 80% tumour cellularity for AK/PAPs and cuSCCs. The chronically UVR-exposed samples from both patients (NS) and mice (CHR) exhibited clear histologic evidence of solar damage including elastosis, fibrosis and chronic inflammation ( Fig. 1 ). Mutational analysis Exome sequencing (Illumina Hi-Seq) was performed on a subset ( Table 1 ) of collected samples with an average coverage of 135 × ±22 (mean±s.d.). The mutational load varied widely across our cohort of well-differentiated primary cuSCC, averaging 2,927 somatic variants (range 385–9,156) or 45.7 variants per Mb ( Fig. 2a ), which is congruent with previously reported results of about 50 mutations per Mb for cuSCC [32] , [33] , [34] , [35] , keeping in mind that some AKs and cuSCCs were referenced to UVR-exposed peri-tumoural NS and not germline ( Table 1 ). AKs had substantially fewer variants, with an average of 1,186 variants (range 290–1,873) or 18.5 per Mb. 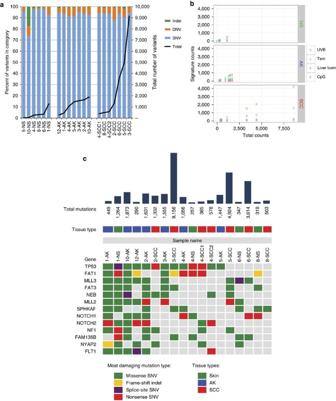Figure 2: The spectrum of mutations in human samples is dominated by C toT transitions and show increasing mutation burden across cuSCC development. (a) cuSCC display very high mutational loads of 45.7 variants per Mb, with NS and AK samples harbouring an average of 5.8 and 18.5 variants per Mb, respectively. There are strongly dominated by single nucleotide variants. (b) NMF-derived orthogonal mutational profiles derived from over 6,000 human cancers confirm a strong enrichment for CpG-associated C→T transitions classically associated with UVB exposure, particularly for AK and cuSCC. For each lesion, the proportion of mutations attributable to a specific signature is plotted as a function of total mutation counts. This correlates strongly with the increasing mutational burden observed in AK and cuSCC, suggesting that the increase is attributable solely to UVB exposure. Three other profiles dominated by C→T transitions are significantly represented in the mutational data and relatively enriched in NS, including ones first described in the context of temozolamide exposure (Tem), one attributed to liver toxins, and one associated with CpG sites. These latter two signatures likely reflect background mutational processes in this context. (c) SMG from this cohort, match those identified previously studied cohorts of cuSCC. Figure 2: The spectrum of mutations in human samples is dominated by C toT transitions and show increasing mutation burden across cuSCC development. ( a ) cuSCC display very high mutational loads of 45.7 variants per Mb, with NS and AK samples harbouring an average of 5.8 and 18.5 variants per Mb, respectively. There are strongly dominated by single nucleotide variants. ( b ) NMF-derived orthogonal mutational profiles derived from over 6,000 human cancers confirm a strong enrichment for CpG-associated C→T transitions classically associated with UVB exposure, particularly for AK and cuSCC. For each lesion, the proportion of mutations attributable to a specific signature is plotted as a function of total mutation counts. This correlates strongly with the increasing mutational burden observed in AK and cuSCC, suggesting that the increase is attributable solely to UVB exposure. Three other profiles dominated by C→T transitions are significantly represented in the mutational data and relatively enriched in NS, including ones first described in the context of temozolamide exposure (Tem), one attributed to liver toxins, and one associated with CpG sites. These latter two signatures likely reflect background mutational processes in this context. ( c ) SMG from this cohort, match those identified previously studied cohorts of cuSCC. Full size image To our surprise, the clinically normal, chronically UVR-exposed skin of patients harboured an average of 372 somatic variants (range 23–1,264) across the exome when referenced to germline DNA samples obtained from saliva, corresponding to an average of 5.8 variants per Mb ( Fig. 2a ). This indicates that the skin sustains substantial mutagenic insults in the course of chronic UVR exposure, as recently reported in UVR-exposed eyelid skin [36] . TP53 mutations have been described before in UVR-exposed skin; however it was not known if this represented ongoing selection specifically for TP53 mutation [37] . Hi-depth targeted sequencing of 74 genes has demonstrated an estimated five mutations per Mb in chronically UVR-exposed eyelid skin, with a strong preponderance of NOTCH1-3, TP53 and FGFR3 mutations suggesting positive selection for these mutations [36] . The spectrum of mutations is very strongly dominated by transitions between cytosine and thymine, in particular from cytosine to thymine (C→T) ( Fig. 2b and Supplementary Figs 1,2a,b ). The proportion of dinucleotide variants that are CC→TT is 90% for both AK and cuSCC and 84% for NS ( Supplementary Fig. 1 ), also highly reflective of UVB exposure. Given the relative statistical rarity of CpG islands across the human genome, the high proportion of C→T transitions at CpG sites reflects the enhanced susceptibility of methylated CpG to deamination and to photoproduct formation [38] . By using non-negative matrix factorization (NMF) -based spectral deconvolution, 21 mutation signatures were derived from over 6,000 specimens across 32 cancer types profiled in TCGA [39] . Three signatures predominated in our samples, which were strongly enriched for C→T transitions ( Fig. 2b and Supplementary Fig. 2a,b ). AK and cuSCC are clearly driven by UVR exposure, with substantial enrichment for the classic UVB C→T transition signature at dipyrimidines [38] in a manner that correlated with increasing mutational load ( Fig. 2b ). NS samples had more evenly represented mutation signatures, including those associated with liver toxin exposure, temozolamide (Tem) exposure and CpG sites ( Fig. 2b and Supplementary Fig. 2a,b ). To identify significantly mutated genes (SMG), we identified those that were recurrently mutated in at least seven pairings and that were either previously implicated in cuSCC or have COSMIC frequencies over 400 ( Fig. 2c and Supplementary Data 1 ). These included genes found to be mutated in metastatic and aggressive cuSCC ( Fig. 2c ) [32] , [33] , [34] , [35] , most prominently, TP53 , NOTCH1-2 , FAT1 and MLL2 . We also identified a rare KNSTRN missense mutation (resulting in p.P28S) in only two pairings (one cuSCC, AK), which appears to be within the same functional domain as a previously reported hotspot p.S25F (ref. 40 ). Importantly, AKs not only have mutations in all of the known SMGs, but AKs have the ‘greatest’ proportion of SMGs represented. This is consistent not only with the notion that AKs have acquired the mutational events necessary for cuSCC formation, but that AKs may harbour multiple clones that have the capacity to ultimately give rise to cuSCC ( Fig. 3a ). There is significant overlap in these variant allele frequency profiles, as all lesion types span a continuum of distributions with a trend of increasing mutational load reflecting increasing monoclonality in NS and AK samples ( Fig. 3a ). Of note, the NS sample (patient 1) with high variant allele frequencies, has evidence for three TP53 mutations ( Fig. 3b ) highlighting how significant mutational loads can be acquired even in the absence of evident dysplasia. Given that mutations exist in hundreds of clones within UVR-exposed skin [36] ( Fig. 2a ), our data suggest that dominant clones may be emerging in AK and cuSCC, particularly in the latter ( Fig. 3a and Supplementary Fig. 3 ), although this sample size was limited. 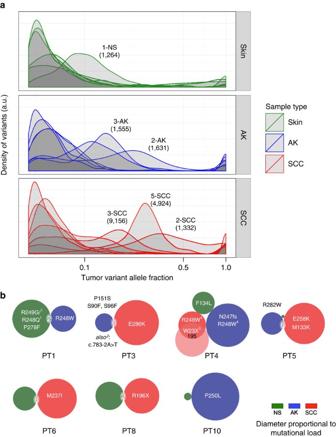Figure 3: Significant mutational heterogeneity and overlap exists between AK and cuSCC. (a) Histograms of variant allele frequencies in NS, AK and cuSCC, show that NS have a large number of low-frequency variants. AK and cuSCC have a more heterogeneous distribution of variant frequencies, with higher-frequency variants, indicative of a general towards the emergence of dominant clones. Outliers with high frequencies of mutations in the NS and AK groups (labelled by patient #) are annotated with mutation frequencies in parentheses to show how these frequencies correlate with increasing monoclonality. (b) Point mutations inTP53compared with overall mutation counts and site-specific ovelaps. Specific mutations are indicated in text, size of the circle indicates the total number of mutations of that sample, with overlaps >1 shown between lesions. R248 is the only amino acid changed in multiple samples within patients 1, 4. Notes regarding specific findings: 1: complex variant at R248/9 hotspot; 2: splice-site variant, 3: appears in both SCC-1 and SCC-2, 4: base change differs between AK and SCC-1 (c.GG741AA in AK, and c.C742T in SCC-1). Figure 3: Significant mutational heterogeneity and overlap exists between AK and cuSCC. ( a ) Histograms of variant allele frequencies in NS, AK and cuSCC, show that NS have a large number of low-frequency variants. AK and cuSCC have a more heterogeneous distribution of variant frequencies, with higher-frequency variants, indicative of a general towards the emergence of dominant clones. Outliers with high frequencies of mutations in the NS and AK groups (labelled by patient #) are annotated with mutation frequencies in parentheses to show how these frequencies correlate with increasing monoclonality. ( b ) Point mutations in TP53 compared with overall mutation counts and site-specific ovelaps. Specific mutations are indicated in text, size of the circle indicates the total number of mutations of that sample, with overlaps >1 shown between lesions. R248 is the only amino acid changed in multiple samples within patients 1, 4. Notes regarding specific findings: 1: complex variant at R248/9 hotspot; 2: splice-site variant, 3: appears in both SCC-1 and SCC-2, 4: base change differs between AK and SCC-1 (c.GG741AA in AK, and c.C742T in SCC-1). Full size image To assess whether a pattern of mutationally driven progression could be ascertained, we then probed whether mutations overlapped between the three groups of samples. Globally, the number of site-specific mutational overlaps between any two sample classes was extremely low and not likely to be significantly different from chance, though the AK to cuSCC comparison had the majority, averaging 3.4 overlaps versus NS to AK (0.75) and NS to cuSCC (1.8) ( Table 2 ). The most significant degree of site-specific mutational overlap occurred between two cuSCCs from patient 4 ( Table 2 ), which were in close physical proximity ( Fig. 1g ; forearm versus hand), strongly suggesting that these physically distinct tumours arose at least in part from a common clone. When viewed within patients, functionally significant genes were mutated in multiple samples, including TP53 (four patients), FAT1 (three patients) and MLL3 (three patients) ( Supplementary Fig. 4 and Supplementary Table 1 ). Overlaps in AK-cuSCC were the most common even among these genes, suggesting that they are specifically targeted in the development of cuSCC. Table 2 Site-specific mutational overlap. Full size table An illustrative example is provided by TP53 , in which multiple mutations were present ( Fig. 3b ). When placed in the context of overall mutational loads and site-specific overlap ( Fig. 3b ), it is evident that the degree of overlap did not closely correlate with physical proximity ( Fig. 1g —patients 1, 3 and 4 with distant AK versus NS/cuSCC and patients 5, 6, 8 and 10 with nearby AK versus NS/cuSCC). The two cuSCCs from patient 4, which shared the greatest overlap (195), shared a TP53 W23X mutant ( Fig. 3b ). Among all the human tumour samples sequenced, only amino acid R248, which is a mutational hotspot in cuSCC [41] , was multiply altered within two patients (patients 1 and 4). These findings are consistent with the concept that mutations that inactivate tumour suppressor genes are often distributed across the entire coding region and that there has not been a strongly dominant oncogenic mutation identified in cuSCC. Transcriptomic analysis RNA and miRNA-seq were performed on the Illumina Hi-Seq platform to yield an average of 64 million and 6.1 million reads, respectively. No significantly expressed fusion or viral transcripts were detected. A correlation matrix using mRNAs differentially expressed in at least one pairwise comparison demonstrated a clear distinction between NS and cuSCC with AKs interspersed across the spectrum ( Fig. 4a ), a pattern also observed in the corresponding gene-sample heatmap and principal component analysis (PCA) plots across all genes ( Supplementary Figs. 5a,b and Supplementary Data 2 ). This shows that even given uniform histological criteria, there is a spectrum of AK that transcriptomically resembles UVR-exposed NS versus some that resemble cuSCC. Global unsupervised clustering of all expressed genes revealed that across all patient samples, six out of the eight complete sets (with tissue from all three lesion types) show that AK segregate with cuSCC by Pearson correlation, a pattern substantiated by the corresponding gene expression heatmaps ( Fig. 4b ). AK and cuSCC are both significantly enriched to a similar degree over peri-tumoural NS for a 70-gene chromosomal instability signature derived from multiple cancers ( Fig. 4c ), again reinforcing the idea that AKs have acquired key genomic features of invasive cuSCC [42] . 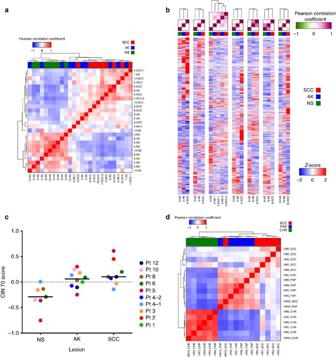Figure 4: mRNA profiling across AK/papilloma and cuSCC development. (a) Correlation matrix of mRNAs differentially expressed in at least one signature in human samples shows that AKs span the spectrum of NS to cuSCC samples. (b) Unsupervised clustering of all genes across patient samples with complete sets (all three lesion types) demonstrates that in 6/8 sets, AK more closely resemble cuSCC. The Pearson correlation matrix is shown on top with the underlying heat map shown below. (c) A 70-gene signature of chromosomal instability derived from human cancers is highly enriched in AK and cuSCC to a similar degree, but not NS. (d) Correlation matrix of mRNAs differentially expressed in at least one signature in mouse samples demonstrates that PAPs much more closely resemble cuSCC than CHR. Figure 4: mRNA profiling across AK/papilloma and cuSCC development. ( a ) Correlation matrix of mRNAs differentially expressed in at least one signature in human samples shows that AKs span the spectrum of NS to cuSCC samples. ( b ) Unsupervised clustering of all genes across patient samples with complete sets (all three lesion types) demonstrates that in 6/8 sets, AK more closely resemble cuSCC. The Pearson correlation matrix is shown on top with the underlying heat map shown below. ( c ) A 70-gene signature of chromosomal instability derived from human cancers is highly enriched in AK and cuSCC to a similar degree, but not NS. ( d ) Correlation matrix of mRNAs differentially expressed in at least one signature in mouse samples demonstrates that PAPs much more closely resemble cuSCC than CHR. Full size image RNA-seq results performed on six sets of samples from Hairless mice corroborated this concept even more strongly, even though they are an outbred strain. Here, the correlation matrix of differentially expressed genes in at least one pairwise comparison clearly delineates CHR away from PAP and cuSCC ( Fig. 4d ), a pattern also observed in the corresponding gene-sample heatmap and PCA plots across all genes ( Supplementary Figs. 5a,c and Supplementary Data 3 ). Next we sought to identify transcription factors that could be responsible for the gene expression changes observed in the course of AK and cuSCC development. Using TRANSFAC-based motif analysis, we identified significantly overrepresented motifs and their associated transcription factors for all pairwise comparisons in both human and mice. Although this method is not unbiased and does not definitively identify biochemical mechanisms of regulation, we surmised that cross-species analysis would enable us to identify significant drivers. First, significant candidate factors were ranked by their enrichment scores ( Supplementary Data 4 ) and selected only if their targets were enriched in genes sets that changed in the same direction for both species in any one of the adjacent pairwise comparisons: NS/CHR to AK/PAP or AK/PAP to cuSCC. These changes also had to be significantly enriched in the NS/CHR to cuSCC comparison. This analysis yielded a total of 17 transcription factors, 11 of which were significant early, and six of which were significant late ( Fig. 5a ). Four factors were globally important across all pairwise comparisons: ETS2, SP1, FREAC2 (FOXF2) and AP1. Gene interaction networks assembled from the overlap of genes predicted to be regulated by multiple transcription factors reveal that these transcription factors are highly interconnected, potentially co-regulating up to several hundred genes in concert ( Fig. 5b ). Though these interactions must be functionally validated in detail, our data suggest that a small core of transcriptional regulators drive cuSCC development. 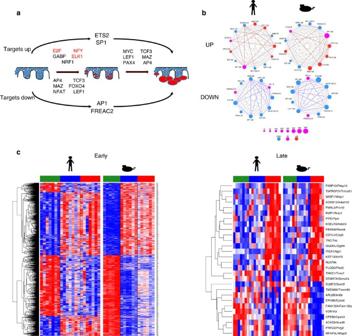Figure 5: Cross-species transcription factor motif analysis reveals major drivers of cuSCC development. (a) Global view of transcription factors with target genes enriched across the entire NS/CHR to AK/PAP to cuSCC progression sequence. Directionality reflects the significant upregulation (above the line) or downregulation (below the line) of predicted targets of the listed transcription factors. Some factors have targets that are enriched in opposite directions across distinct transitions. The transcription factors highlighted in red were identified in both TRANSFAC and LME-based analyses. (b) Network analysis demonstrates that core transcriptional drivers are highly interconnected in both human (left) and mouse (right). The bolded lines delineate connections that are significant by Fisher exact test (P<10−4). (c) The LME model of mRNA expression changes across cuSCC development in both species demonstrates that the vast majority of significant gene expression changes occur in the early transition from NS/CHR to AK/PAP. Figure 5: Cross-species transcription factor motif analysis reveals major drivers of cuSCC development. ( a ) Global view of transcription factors with target genes enriched across the entire NS/CHR to AK/PAP to cuSCC progression sequence. Directionality reflects the significant upregulation (above the line) or downregulation (below the line) of predicted targets of the listed transcription factors. Some factors have targets that are enriched in opposite directions across distinct transitions. The transcription factors highlighted in red were identified in both TRANSFAC and LME-based analyses. ( b ) Network analysis demonstrates that core transcriptional drivers are highly interconnected in both human (left) and mouse (right). The bolded lines delineate connections that are significant by Fisher exact test ( P <10 −4 ). ( c ) The LME model of mRNA expression changes across cuSCC development in both species demonstrates that the vast majority of significant gene expression changes occur in the early transition from NS/CHR to AK/PAP. Full size image Importantly, some transcription factors, such as ETS2, showed largely unidirectional target modulation, but others such as TCF3 and LEF1 had significant target modulation in opposite directions, reflecting transition-specific changes ( Supplementary Fig. 6a–i ). Profiles of the four globally important transcription factors showed significant upregulation of ETS2 and SP1 and downregulation of FREAC2 (FOXF2) and AP1 targets across the entire progression sequence ( Fig. 5a and Supplementary Data 4 ). ETS2 ( Supplementary Fig. 6a ) is pro-oncogenic in multiple other contexts, and is downstream of the ERK MAP kinase signalling module [43] , which is known to be important in sporadic and BRAF-inhibitor-induced cuSCC development [44] , [45] . The global upregulation of SP1 targets ( Supplementary Fig. 6b ) may reflect its ability to partner with a number of transcription factors in cancer [46] . As expected, β-catenin/Wnt signalling plays an important role in cuSCC pathogenesis and this is reflected in the importance in this analysis of both TCF3 and LEF1 activity. TCF3 can function as a transcriptional repressor and activator and has been implicated in skin homoeostasis and wound healing [47] . Our data suggest an important role in cuSCC development as well ( Supplementary Fig. 6c ). LEF1 appears to be activated across the spectrum of samples, with targets significantly downregulated early and upregulated late ( Supplementary Fig. 6d ), and is an established effector of β-catenin/Wnt signaling [48] . The downregulation of NFAT targets early ( Supplementary Fig. 6e ) may reflect an inhibition of keratinocyte differentiation programs that may be modulated by NOTCH signalling and further compromise TP53 -dependent tumour suppression [49] . Similarly, the predicted downregulation of AP1 target genes across the continuum of cuSCC development ( Supplementary Fig. 6f ) suggests a compromise of normal epidermal differentiation [50] . FREAC2 (FOXF2) targets are downregulated across the development sequence ( Supplementary Fig. 6g ), and although it has not been specifically implicated in skin cancer, downregulation of its expression promotes epithelial–mesenchymal transition in basal breast cancer [51] . Consistent with our global transcriptomic data, most of the transcriptional drivers are predicted to act early in the NS/CHR to AK/PAP transition, including NFY, E2F and ELK1, with some, including MYC activation, occurring late ( Fig. 5a and Supplementary Fig. 6h,i ). Both E2F and MYC have been implicated in cuSCC development [44] . Although using individual pairwise analysis suggested key transcriptional regulators, we also used a linear mixed effects (LME) model previously employed to identify differentially expressed genes in matched normal, premalignant and tumour samples from patients with lung SCC (LUSC) [52] . Following cross-species overlap of mouse and human data, this model also clearly demonstrated that the majority of changes occur in the earliest transition from NS to AK/PAP versus the subsequent transition to cuSCC ( Fig. 5c and Supplementary Data 5 ). In GATHER-based analysis of TRANSFAC motifs within concordantly differentially expressed genes [53] by this analysis, E2F and NFY ( Supplementary Fig. 6h,i and Supplementary Data 6 ) were again highlighted in the early stage transition from NS to AK/PAP in both mouse and human. ELK1, which is likewise regulated by the ERK MAPK pathway, was also significant by both analyses ( Fig. 5a and Supplementary Data 6 ). No enriched transcription factor signatures were identified for the late-stage AK/PAP to cuSCC transition using the LME model. On the basis of these sets of differentially expressed genes, Ingenuity Pathway Analysis of both human and mouse data was performed individually ( Supplementary Table 2 ) and identified strongly overlapping key pathways including cell cycle progression, mitotic roles of polo-like kinase and DNA damage checkpoint functions, as well as upstream regulators E2F1, E2F4, CDK4, TP53, RABL6 and ERBB2, the latter two of which may be novel targets for intervention. The transcriptional networks identified in both the pairwise analyses and the progression model analysis implicate pathways important in cuSCC development, mostly early in the NS/CHR to AK/PAP transition, notably E2F, ELK1 and NFY. ERK signalling through ETS2, β-catenin signalling through TCF3 and LEF1, and pathways regulated by NFAT and AP1 that likely impinge upon keratinocyte differentiation, were implicated globally across the entire development sequence ( Fig. 5 ). MicroRNA sequencing and integrated analysis Relative to mRNA, clustering of microRNAs differentially expressed in at least one pairwise comparison among the matched human samples showed a better ability to distinguish the three sample classes ( Fig. 6a ). When recurrent statistically significant changes occurring in at least two out of three pairwise comparisons are used, it is clear that AKs now define a pattern of microRNA expression that is intermediate between NS and cuSCC, with improved discrimination between sample types ( Fig. 6b , Supplementary Data 7 and Supplementary Fig. 7 ). 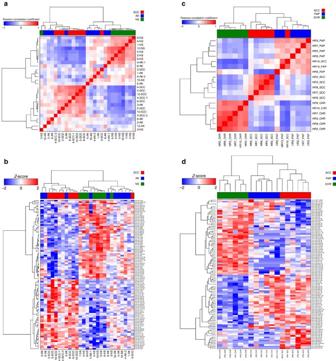Figure 6: microRNA profiling across AK/papilloma and cuSCC development. (a) Correlation matrix of microRNAs differentially expressed in at least one signature in human samples shows that significantly improved discrimination between three sample types is achieved as compared with mRNA profiles. (b) Using only microRNAs differentially expressed in at least two out of three pairwise comparisons (P<0.05), robust discrimination is achieved between NS and cuSCC with most AKs occupying an intermediate expression pattern. (c) Hierarchical clustering of microRNAs differentially expressed in at least one signature in mouse samples shows distinct patterns among the three sample types as compared with mRNA profiles. (d) Using only microRNAs differentially expressed in at least two of three pairwise comparisons (P<0.05), CHR and cuSCC are very strongly segregated with an intermediate group dominated by PAP. Figure 6: microRNA profiling across AK/papilloma and cuSCC development. ( a ) Correlation matrix of microRNAs differentially expressed in at least one signature in human samples shows that significantly improved discrimination between three sample types is achieved as compared with mRNA profiles. ( b ) Using only microRNAs differentially expressed in at least two out of three pairwise comparisons ( P <0.05), robust discrimination is achieved between NS and cuSCC with most AKs occupying an intermediate expression pattern. ( c ) Hierarchical clustering of microRNAs differentially expressed in at least one signature in mouse samples shows distinct patterns among the three sample types as compared with mRNA profiles. ( d ) Using only microRNAs differentially expressed in at least two of three pairwise comparisons ( P <0.05), CHR and cuSCC are very strongly segregated with an intermediate group dominated by PAP. Full size image Whereas unsupervised clustering of mRNA expression in the Hairless mouse model failed to distinguish papillomas from cuSCC ( Fig. 4d ), unsupervised clustering of microRNA expression more clearly separates all three sample types ( Fig. 6c,d , Supplementary Data 8 and Supplementary Fig. 7 ), suggesting that microRNAs have more discriminatory power as compared with mRNA in segregating the sample types. Given that microRNAs can negatively regulate their target mRNA expression by Watson-Crick pairing over a 7–8 nucleotide seed region, we performed functional pair analysis by identifying miRNA–mRNA pairs predicted to be linked by a seed sequence in the 3′UTR of the mRNA and that were significantly anti-correlated in expression changes [54] . Functional pairs in both species were ranked by all possible pairwise comparisons in which they were significantly differentially expressed (rather than by stage), and an integrated network map was generated to identify several key microRNAs with multiply targeted mRNAs ( Fig. 7a,b ). 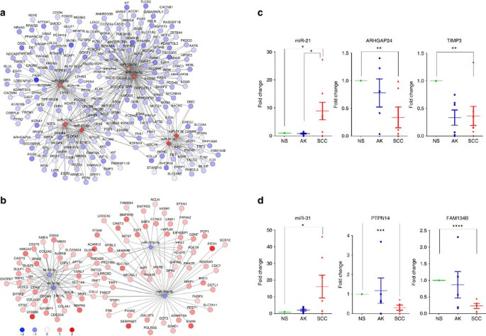Figure 7: Functional pair analysis identifies highly interconnected microRNA/mRNA regulatory networks conserved across species. This occurs for both (a) upregulated microRNAs/downregulated target mRNAs and for (b) downregulated microRNAs/upregulated target mRNAs. The figures only show those microRNAs withq<10−8, log2-fold change of >1.15, conserved between species. Validation of select microRNA/mRNA pairs using a distinct set of human matched samples demonstrate robustness of the findings. (c) miR-21 is upregulated between NS and cuSCC, whereas predicted targets ARHGAP24 and TIMP3 are downregulated. (d) miR-31 is upregulated between NS and cuSCC, whereas predicted targets PTPN14 and FAM134B are downregulated. Figure 7: Functional pair analysis identifies highly interconnected microRNA/mRNA regulatory networks conserved across species. This occurs for both ( a ) upregulated microRNAs/downregulated target mRNAs and for ( b ) downregulated microRNAs/upregulated target mRNAs. The figures only show those microRNAs with q <10 −8 , log 2 -fold change of >1.15, conserved between species. Validation of select microRNA/mRNA pairs using a distinct set of human matched samples demonstrate robustness of the findings. ( c ) miR-21 is upregulated between NS and cuSCC, whereas predicted targets ARHGAP24 and TIMP3 are downregulated. ( d ) miR-31 is upregulated between NS and cuSCC, whereas predicted targets PTPN14 and FAM134B are downregulated. Full size image The microRNAs significantly upregulated in this cross-species analysis included miRs-15a/b, 17, 20a, 21, 31, 200a and 340b ( Fig. 7a ), and those significantly downregulated included let-7 family members and miRs-30a and 125b ( Fig. 7b ). Some of these microRNAs are confirmed in our data to be significant in cuSCC. miR-21 and miR-31 have been shown to be upregulated in a number of cancers including cuSCC [55] , [56] , [57] , although the identity of the most relevant mRNA targets is not known. In many instances, functionally paired mRNAs were predicted to be targeted by multiple microRNAs. We validated the expression levels of miR-21 and miR-31 and of selected predicted target genes in additional sets ( n =21) of matched human samples of NS, AK, and cuSCC ( Fig. 7c,d and Supplementary Data 9 ). miR-21 was substantially upregulated by 8.9±3.1-fold (mean±s.e.m. ; n =8 sets) across the progression sequence, with respective downregulation of the predicted targets ARHGAP24 (2.9±0.6-fold; mean±s.e.m. ; n =6 sets) and TIMP3 (3.0±0.4-fold; mean±s.e.m. ; n =6 sets) ( Fig. 7c ). ARHGAP24 is a RAC1 GAP (ref. 58 ), and TIMP3 suppresses metalloproteinase function, both of which are consistent with tumour suppressive functions. miR-31 was also upregulated (16.2±6.8-fold; mean±s.e.m. ; n =7 sets) across cuSCC development and predicted to downregulate PTPN14 (3.2±0.4-fold; mean±s.e.m. ; n =5 sets), a phosphatase which downregulates YAP signalling [59] ( Fig. 7d ). In addition, FAM134B, a putative tumour suppressor [60] was identified as a potential target of miR-31 (down 4.3±1.4-fold; mean±s.e.m. ; n =5 sets; Fig. 7d ). The let-7 family of microRNAs is prominently represented among downregulated microRNAs, consistent with a tumour suppressor role, and one of the predicted targets, HMG2A, was substantially upregulated in a validation cohort by 45.4±14.5-fold (mean±s.e.m. ; n =4 sets). These specific pairs need to be functionally validated to provide mechanistic links, but these data show that the cross-species functional pair analysis is robust. Relationship of cuSCC to other SCC Many types of SCC arising in diverse sites, such as lung, oesophagus, bladder, cervix and head and neck SCC (HNSCC) have now been genomically profiled, in addition to exome sequencing of cutaneous SCC [32] , [33] , [34] , [35] . These combined efforts have collectively identified common pathway alterations for many SCCs. TP53 mutations occur at over 70% frequency in all SCCs; NOTCH family genes are mutated in over 70% of cuSCC [32] , [33] , 10–20% of HNSCC [61] , [62] , [63] , 13% of LUSC [64] and 10% of oesophageal SCC (ESCA SCC) [65] ; and SOX2 amplification is a common lineage-specific driver of SCC [66] . To test the hypothesis that mRNA expression profiles would reveal molecular commonalities between all SCC, we profiled our NS/cuSCC signature against cancers in the TCGA using gene set enrichment analysis (GSEA). Furthermore, we surmised that there would be major differences between carcinogen-driven versus virally driven SCC, as observed in HNSCC [61] , [62] , [63] . We found that cuSCC is most similar to HNSCC, followed by LUSC, basal (triple-negative) and HER2 breast cancer and ESCA SCC, but not closely related to cervical SCC, which is overwhelmingly human papillomavirus (HPV) -driven ( Fig. 8a and Supplementary Data 10 ). This establishes transcriptomic evidence that deep molecular commonalities exist between carcinogen-driven SCCs of multiple tissue sites, a concept supported by the mutational data, and suggests that common molecular strategies for prevention and treatment of multiple types of SCCs may exist. 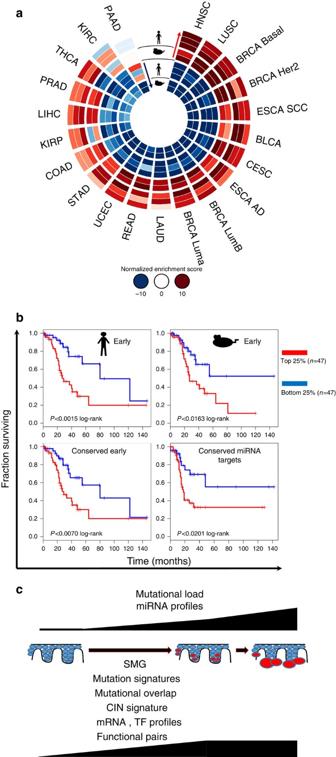Figure 8: cuSCC is molecularly related to carcinogen-driven SCCs of multiple sites. (a) GSEA analysis of all significant pairwise comparisons in both mouse (CHR versus PAP, CHR versus cuSCC) and human (NS versus AK, AK versus cuSCC, NS versus cuSCC) represented as a CIRCOS plot. For all cancers profiled in the TCGA, normalized enrichment scores for each signature were determined and cancer types ranked by descending order (clockwise) of the sum of squares of all the scores with a penalty. By this measure, cuSCC is most closely related to HNSC, LUSC, basal and HER2+ subtypes of breast cancer (BRCA) and ESCA SCC. (b) Given that HNSC is most closely related to cuSCC by this measure, we show that cuSCC signatures can predict outcome (overall survival) in HNSC withTP53mutation, used here as a proxy for identifying tumours that do not express high-risk HPV. The cross-species early signatures derived from the linear mixed effects model and the cross-species microRNA functional analysis all predict survival in HNSCC for the top and bottom 25% of outcomes with statistical significance. Multiple hypothesis testing was performed and all of the plots shown are significant with the statedP-values and false discovery rate-adjustedq-values of <0.1 (q=0.021 human early, 0.070 mouse early, 0.049 conserved early and 0.070 conserved miRNA targets). (c) Taken together, our data show that AKs have acquired many of the properties of cuSCC as assessed by SMG, mutational overlap, mutational signatures, chromosomal instability signature, mRNA and transcription factor profiles and functional pair analysis, although overall mutational load and unsupervised microRNA clustering do enable separation of the three sample types. Figure 8: cuSCC is molecularly related to carcinogen-driven SCCs of multiple sites. ( a ) GSEA analysis of all significant pairwise comparisons in both mouse (CHR versus PAP, CHR versus cuSCC) and human (NS versus AK, AK versus cuSCC, NS versus cuSCC) represented as a CIRCOS plot. For all cancers profiled in the TCGA, normalized enrichment scores for each signature were determined and cancer types ranked by descending order (clockwise) of the sum of squares of all the scores with a penalty. By this measure, cuSCC is most closely related to HNSC, LUSC, basal and HER2+ subtypes of breast cancer (BRCA) and ESCA SCC. ( b ) Given that HNSC is most closely related to cuSCC by this measure, we show that cuSCC signatures can predict outcome (overall survival) in HNSC with TP53 mutation, used here as a proxy for identifying tumours that do not express high-risk HPV. The cross-species early signatures derived from the linear mixed effects model and the cross-species microRNA functional analysis all predict survival in HNSCC for the top and bottom 25% of outcomes with statistical significance. Multiple hypothesis testing was performed and all of the plots shown are significant with the stated P -values and false discovery rate-adjusted q -values of <0.1 ( q =0.021 human early, 0.070 mouse early, 0.049 conserved early and 0.070 conserved miRNA targets). ( c ) Taken together, our data show that AKs have acquired many of the properties of cuSCC as assessed by SMG, mutational overlap, mutational signatures, chromosomal instability signature, mRNA and transcription factor profiles and functional pair analysis, although overall mutational load and unsupervised microRNA clustering do enable separation of the three sample types. Full size image Given that HNSCC is consistently the most closely related tumour to cuSCC, we asked whether cuSCC-derived signatures from our cohort of well-differentiated tumours could also be used to predict outcomes in carcinogen-driven (non-HPV) HNSCCs, which have TP53 mutations and high mutational loads [63] . When we restricted the cuSCC signatures to early genes identified in the LME progression model for either human or mouse independently ( Fig. 5c ), both signatures were significantly predictive of overall survival ( Fig. 8b —top row). Similarly, when we used only the cross-species intersection of these two signatures of early genes, this was again significantly predictive of overall survival ( Fig. 8b —bottom left, Supplementary Fig. 8 ). Most importantly, a 309-gene signature derived solely from the cross-species microRNA functional pair analysis ( Fig. 7a,b ) had significant predictive power for overall survival ( Fig. 8b —bottom right), showing that these microRNA target genes likely regulate not only important processes in cuSCC development but also drivers of disease outcome in HNSCC. Our analysis is the first comprehensive characterization of genomic changes that drive the development of cuSCC through its preneoplastic intermediate, the AK, employing the combination of matched human patient samples, next-generation sequencing, and cross-species analysis. Despite the clear clinical and histological distinctions between cuSCC, AK and perilesional UVR-damaged skin, AK/PAP are most closely related to cuSCC, by many measures including mRNA expression (unsupervised clustering and LME model), transcription factor motif analysis, mutational signatures and overlap, chromosomal instability signature expression, and microRNA–mRNA functional pair analysis ( Fig. 8c ). Our data confirm the high mutational burden of these skin cancers [32] , [33] , [34] , [35] . Importantly, high mutational loads have recently been described in chronically UVR-exposed blepharoplasty samples [36] , and, for the first time, we show the large degree of mosaicism present across the entire exome in non-lesional UVR-exposed peri-tumoural skin, with quantitatively similar mutational loads ( Fig. 2 ). The SMGs identified, including TP53 , NOTCH1-2 , FAT1 and MLL2 are ones likely to be important in cuSCC pathogenesis ( Fig. 2c ) [32] , [33] , [34] , [35] . Conversely, one of the most frequently mutated genes previously identified in sun-exposed skin, FGFR3 , was not found to be mutated, suggesting that this genetic lesion, frequently found in seborrheic keratoses, may be specifically critical for benign keratoses and not non-melanoma skin cancers [36] . Our findings are consistent with the notion that tumour suppressor genes, which represent the largest class of cancer genes known to be recurrently targeted in cuSCC, can often be inactivated by mutational insults spread across their entire coding regions. The overwhelming preponderance of epidemiological, clinical and biological data suggest that UVR exposure is the main driver of sporadic cuSCC development. The subsequent expansion in overall mutational load, which occurs in progression to AK and cuSCC correlates with a significant enrichment for UVB-signature mutations ( Fig. 2b ). It is possible that this is reflective of a progressively more clonal structure across the continuum from NS to AK to cuSCC, although our sample size is small ( Fig. 3a ). The lower relative representation of the UVB signature in the NS samples maybe due to low sensitivity for detecting small subclones induced by UVR exposure at a given sequencing depth ( Fig. 2b ). It is possible that initiated clones persist longer than normal keratinocytes, thereby enabling expansion or accumulation of further UVB-mediated DNA damage, a notion consistent with the early appearance of TP53 mutations ( Figs 2c and 3b ) [36] , and dramatically illustrated in the NS sample from patient 1 ( Figs 2a,b and 3b ). Other contributory mechanisms could include compromised DNA repair, compromised photoprotection by melanocytes, or the generation of these types of mutations in the absence of UVR exposure. Finally, the overlap in specific mutations was low ( Fig. 3b , Table 2 ) and while this may also be due to the inability to detect small subclones particularly in the NS and AK samples, all the lesions (particularly AKs) were physically distinct. Nevertheless, the dramatic overlap in mutations between the two separate SCCs in patient 4 strongly suggests that clones of UVR-initiated keratinocytes can populate large areas of epidermis ( Fig. 3b and Table 2 ). SCCs arise at interfaces with the environment, thus making them susceptible to sustained carcinogenic insults. Our data support the notion that cuSCC, HNSCC, LUSC and ESCA SCC share deep molecular commonalities ( Fig. 8a ) at the mutational and transcriptional levels, and include deregulation of key pathways such as those driven by altered RB1 , TP53 and TP63 function [32] , [34] , [35] , [63] , [64] , [65] . Therefore, for the subsets of these SCCs driven by UVR, alcohol and tobacco exposure, common molecular treatment and prevention strategies may potentially be developed and modelled on cuSCCs, which are substantially more accessible and common. The unexpected molecular similarity of cuSCC to specific subtypes of breast cancer may also highlight similar molecular vulnerabilities such as ERBB2/HER2 ( Fig. 8a and Supplementary Table 2 ). Interestingly, there was much less similarity between cuSCC and cervical SCC ( Fig. 8a ). cuSCC does not appear to require HPV transcription for tumour maintenance, whereas cervical SCC is overwhelmingly driven by high-risk αHPV infection [67] . While AKs appear already to harbour the majority of events that are retained in cuSCC, at least two alternative explanations are possible: (1) consistent mutational or transcriptomic events that separate AKs versus cuSCC could be present, and/or (2) there are distinct molecular classes of AKs with different risks of progression to cuSCC. Either of these explanations would require much larger numbers of samples to demonstrate. Nevertheless, our data show that microRNA expression distinguishes the three sample classes and may potentially serve as a basis for distinguishing different types of AKs ( Fig. 6 ). In addition, our cross-species functional pair analysis has identified a handful of highly interconnected microRNA–mRNA networks that drive cuSCC development through preneoplastic AKs ( Fig. 7 ), highlighting specific microRNA targets for potential intervention. Nevertheless, given the many significant similarities between AK and cuSCC, our data suggest that non-lesional carcinogen-exposed fields of tissue may represent the most effective point of intervention for molecularly targeted chemoprevention. The development of cancer through a preneoplastic intermediate has been studied extensively in Barrett’s oesophagus and oesophageal adenocarcinoma [68] , [69] . Barrett’s oesophagus that evolves into adenocarcinoma can be largely indistinguishable from carcinoma, consistent with our conclusion that for a subset of patients, field-based treatment is most appropriate. AKs are typically too small to allow for repeated sampling, thus removing the possibility for longitudinal follow-up and clinical discernment between AKs that ultimately progress and those that do not. Nevertheless, it is likely that AKs are polyclonal reservoirs from which cuSCCs can arise ( Fig. 3a ), and it is unclear whether catastrophic genomic instability drives this late transition. Our data substantiate the power of cross-species analysis to identify biologically important pathways in cuSCC development and suggests that the solar UVR-exposed Hairless mouse model is a useful testbed for chemopreventive and treatment modalities. Other mouse models of cuSCC have also been extensively studied, most prominently the DMBA/TPA model [70] ; in this model, tumorigenesis is overwhelmingly driven by Hras Q61 mutations which are rarely found in UVR-driven human cuSCC and in the UVR-driven Hairless mouse model ( Supplementary Data 1 ) [24] , [32] , [33] , [34] , [35] . The key transcriptional drivers we identified in both pairwise signatures and the LME model are important early in the NS/CHR to AK/PAP transition and include E2F, ELK1 and NFY. Globally, we identified ERK signalling through ETS2 and ELK1, β-catenin signalling through TCF3 and LEF1, and possible differentiation pathways regulated by NFAT and AP1 as potentially important drivers of cuSCC development ( Fig. 5 ). The significant enrichment of signatures from both patient samples and the UVR-driven Hairless model in multiple carcinogen-driven SCCs arising in diverse sites is important in that it establishes the concept that these SCCs are molecularly closely related ( Fig. 8a ). Furthermore, early cuSCC signatures were able to predict survival in TP53 -mutant (non-HPV) HNSCC ( Fig. 8b ). This suggests that a common set of biological processes underlie the development of multiple SCC types, and that cuSCC may serve as an accurate and extremely accessible model for exploring pathogenesis and testing interventions. Human tissue samples All human tissues were studied under a MD Anderson Cancer Center IRB-approved protocol (LAB08-0750). All human tissues were obtained from patients who provided written informed consent and who had no history of immunosuppression. These samples were validated by histological analysis and processed using standard methods to yield both high-quality DNA and RNA (RIN>8.0). Mouse model of UVR-driven cuSCC All mouse studies were conducted under MD Anderson Cancer Center IACUC-approved protocol (ACUF 00001396-RN00). Mice were obtained from Charles River Laboratories. To model UVR-driven cuSCC under controlled conditions, we exposed female SKH1-E Hairless mice to chronic low-dose UVR (12.5 kJ m −2 UVB total weekly divided in three doses M, W, F) using solar simulators (Oriel) starting at 3 months of age. In this strain, 5.0 kJ m −2 UVB is ∼ 0.5–1 mean erythemal dose [71] . These mice lack the Hairless gene, and they are highly susceptible to UVR-induced skin tumours, UVR-induced immunosuppression and DNA damage [23] . In our studies, we have used solar simulators with well-characterized spectra at 2.5–5.0 kJ m −2 UVB 3 days a week for a total of 12.5 kJ m −2 per week (275–325 nm) (ref. 71 ). These doses were verified by broadband UVB and ultraviolet A (UVA) measurements (ILT1700/ILT73B) in experimental conditions before this experiment. Doses of UVB and UVA averaged 12.5 and 145 kJ m −2 weekly, respectively. In this model of UVR-driven cuSCC development, we irradiated the mice for 100 days. Papillomas were typically observed within this time and were histologically well-differentiated. A minority of these lesions to invasive well-differentiated cuSCC. Preparation of RNA for illumina sequencing Tissue specimens (50–200 mg) were homogenized with an Omni rotor stator homogenizer in TRIZOL (Invitrogen Cat # 15596018). Total RNA was extracted according to the manufacturer instructions. RNA purification was carried with Purelink RNA kit (Invitrogen Cat #12183018A). 4–10 μg of RNA per sample was submitted for 76 nt paired-end sequencing by lllumina HiSeq 2000. The same samples were submitted to the laboratory of Preethi Gunaratne, PhD (University of Houston, Biology & Biochemistry) for small RNA sequencing. DNA isolation and exome seq PureLink Genomic DNA mini kits were used to extract DNA from tissue samples (Cat # K1820-01). Briefly, tissue specimens were minced and incubated overnight (55 °C) in PureLink genomic digestion buffer and proteinase K. Manufacturer’s protocol was followed for purification using the spin columns. Two microgram of DNA per sample was submitted to MD Anderson DNA Analysis Facility for sequencing (Illumina HiSeq200, 76 nt PE). We used DNA Genotek ORAgene saliva collection kits and followed manufactures’ collection and storage instructions (catalogue # OG-500). Genomic DNA was isolated from saliva samples using DNA Genotek prepIT·C2D (PT-C2D) extraction columns and manufacturers’ protocol. Exome analysis For any given patient, if their saliva samples were available, they were used as the paired control for the mutation detection. Otherwise, NS samples were used as controls. Four precapture libraries were pooled together and hybridized according to the manufacturer’s protocol NimbleGen SeqCap EZ Exome Version 3. Exomes were sequenced on an Illumina HiSeq 2000 platform to an average coverage of 135X. Sequencing runs generated approximately 300–400 million successful reads on each lane of a flow cell, yielding 9–12 Gb per sample. Initial sequence analysis was performed using the HGSC Mercury analysis pipeline ( https://www.hgsc.bcm.edu/software/mercury ). First, the primary analysis software on the instrument produces.bcl files that are transferred off-instrument into the HGSC analysis infrastructure by the HiSeq Real-time Analysis module. Next, the vendor’s primary analysis software (CASAVA) demultiplexes pooled samples and generates sequence reads and base-call confidence values (qualities). Reads are mapped to the GRCh37 Human reference genome ( http://www.ncbi.nlm.nih.gov/projects/genome/assembly/grc/human/ ) using the Burrows-Wheeler aligner (BWA, http://bio-bwa.sourceforge.net/ ) and producing a BAM file. Finally, quality is recalibrated (GATK, http://www.broadinstitute.org/gatk/ ), and separate sequence-event BAMs are merged into a single-sample-level BAM. BAM sorting, duplicate read marking, and realignment to improve in/del discovery all occur at this step. Mutations were identified by using the HGSC Cancer Genomics pipeline which includes variant calling using Atlas-SNP, Atlas-INDEL, and PInDel on each of the BAM files and then merging the variant calls and performing allele lookups. Merged variant files were annotated using dbSNP, COSMIC and Annovar and then split into somatic and germline calls based on variant quality and segregation. Variant calls were then filtered using a cohort filtering approach and filtered variants were analysed. DNPs were collapsed with their neighbours and annotated by using Provean (provean.jcvi.org). Identification of SMGs essentially paralleled our previously established pipeline [34] . Non-negative matrix factorization-based mutation signatures NMF-based spectral deconvolution was used to derive signatures based upon mutations placed in trinucleotide context. The method used is mathematically similar to one recently applied to similar cancer data sets [72] , but has the advantage of removing the partial overlap between the reported signatures that resulted in high correlations between some of them [39] . Our strategy employed non-smooth NMF, a variant, which approximates the data using the basis and coefficient matrices as above with the addition of a third smoothing matrix which serves to absorb noise within the data, thus driving the coefficient and basis matrices to increase sparseness. The resulting basis matrix generated k =21 signatures from a diverse set of over 6,000 cancers [39] , reducing correlations between signatures originally derived by Alexandrov et al . [72] thereby increasing orthogonality. This enhanced orthogonality has the potential advantage of suggesting biological mechanisms of mutation generation with greater specificity. RNA-Seq analysis RNA sequencing (Illumina Hi-Seq) yielded 30–40 million read pairs for each sample. The mRNA-seq paired-end reads were aligned to the human reference genome, GRCh37/hg19, using the MOSAIK alignment software [73] . The mRNA-Seq mouse sample reads were aligned onto the mouse genome build UCSC mm10 (NCBI 38). The overlaps between aligned reads and annotated genomic features, such as genes/exons were counted using the HTSeq software platform ( http://www-huber.embl.de/users/anders/HTSeq/doc/overview.html ). The counts were normalized using the scaling factor method. To perform further analysis, the normalized counts were transformed by the variance-stabilizing transformation method and were corrected for experimental batch effects. Specifically, the median expression of each batch was scaled to the same value per gene. Hierarchical clustering analysis, using the Pearson correlation coefficient as the distance metric, complete linkage, and PCA were performed using the R statistical system ( https://www.r-project.org ). Genes significantly differentially expressed between the NS/CHR, AK/PAP, and cuSCC stages were determined using the R package DESeq2 (ref. 74 ). Since multiple genes were tested simultaneously, the Benjamini-Hochberg method was used to control false discovery rate. For further integration of mRNAs and miRNAs, and detection of enriched transcription factor targets, we used a cutoff of Q -value<0.25 and fold-change exceeding 1.25 × . Viral and fusion transcripts were assessed using the VirusSeq algorithm [75] given that mapping viral integration sites is computationally similar to identifying fusion events. In brief, non-human reads were aligned to viral sequences from the Genome Information Broker for Viruses ( http://gib-v.genes.nig.ac.jp/ ) with overall counts registered. Discordant paired-end reads that support a fusion event were clustered and the candidates reported using supporting pairs (at least four) and junction spanning reads (at least one) as the cut-offs. TRANSFAC-based analysis ( http://www.gene-regulation.com/index2.html ) was performed by first identifying significantly overrepresented motifs and their associated transcription factors for all pairwise comparisons in both human and mice. First, significant candidate factors were ranked by their enrichment scores ( Supplementary Data 4 ) and selected only if their targets were enriched in genes sets that changed in the same direction for both species in any one of the adjacent pairwise comparisons: NS/CHR to AK/PAP or AK/PAP to cuSCC. These changes also had to be significantly enriched in the NS/CHR to cuSCC comparison. To quantify chromosomal instability (CIN), CIN70 score was calculated by summing up the normalized counts of all CIN70 genes [42] . To adjust the effects of multiple samples per patient and experimental batches, CIN70 scores were first transformed by the variance-stabilizing transformation method implemented in DESeq2 and fit into a linear model with patients and experimental batches as covariates. The residuals of the linear model were treated as adjusted CIN70 scores. Cross-species linear mixed effects model This analysis was confined to human samples that had complete matched sets of lesion types (21 samples from six patients). Samples from all six mice were used. For each gene, LME models were constructed in which normalized gene expression (as above) was modelled as a function of sample type (fixed effect) while correcting for the patient or mouse source (random effect). The models were created twice, using either NS/CHR or AK/PAP as the reference group to compute coefficients, and t tests were performed to assign significance to each gene with respect to each coefficient in each model. From those genes for which both iterations of the model were successfully fitted to the data (numerically stable), a set of genes with nominal P <0.05 for the cuSCC versus NS/CHR coefficient was identified. Each of these sets was then filtered to identify genes for which the AK/PAP versus NS/CHR or the cuSCC versus AK/PAP coefficient also had a nominal P <0.05 and a sign matching that of the cuSCC versus NS/CHR coefficient; these genes were designated as early and late, respectively, or stepwise (both early and late). LME modelling and t tests were carried out using the R package v.3.1-97 (( https://www.r-project.org ). For cross-species analysis, the NCBI HomoloGene resource (version 68) ( http://www.ncbi.nlm.nih.gov/homologene ) was used to facilitate cross-species analysis as follows. First, HUGO identifiers were converted to Entrez Gene identifiers. Most (>95%) of the identifiers could be translated in this manner (16,155 out of 16,952 human features and 14,084 out of 14,542 mouse features); features that did not map to an Entrez Gene ID were discarded. Next, the resulting Entrez Gene identifiers were matched between species by common HomoloGene identifier, and any feature from either data set that did not map to exactly one homologue in the other data set was discarded. Finally, the LME results from the two data sets were merged by HomoloGene identifier to allow for direct comparison. GATHER (Gene Annotation Tool to Help Explain Relationships) [53] was used to identify TRANSFAC identifiers that were significantly overrepresented in the early (NS/CHR to AK/PAP), late (AK/PAP to cuSCC), and stepwise (both early and late) gene sets, with a Bayes Factor >3 considered significant. smallRNA-Seq analysis This work was performed with collaboration with laboratory of Dr Preethi Gunaratne, PhD (University of Houston, Biology & Biochemistry). Illumina small RNA adapter sequences were trimmed from the reads, and reads of length below 10nt or ending in homopolymers of length 9 nt or above were discarded. Total usable number of reads for each sample was calculated. The reads were mapped to the miRBase [76] reference ( http://www.mirbase.org/ ) using BLAST; the abundance of each expressed microRNA was quantified as a fraction of the usable reads, and expressed as parts per million To reduce potential batch effects due to sample collection and preparation at different times, the ComBat normalization algorithm [77] ( http://www.bu.edu/jlab/wp-assets/ComBat/Abstract.html ) was applied for the human data. We determined differentially expressed microRNAs imposing a fold-change of 1.5 × and t -test comparison ( P <0.05) using the R statistical system. We employed PCA to examine sample structure; further visualization of microRNA significant in one or multiple comparisons was carried out using the R statistical system. Integrative mRNA-miRNA functional pair analysis We determined enriched miRNA–mRNA pairs using the SigTerms methodology. Essentially, by applying a one-sided Fisher exact test and using TargetScan [78] ( http://www.targetscan.org/vert_71/ ) predicted microRNA targets, we determined the miRNAs for which the gene targets are significantly enriched (false discovery rate-adjusted q <0.25; fold-change>1.25 × ) in the gene signature, separately for the human specimens and the mouse samples. Finally, we determined the conserved enriched miRNAs alongside the SCC progression model, and the conserved miRNA–mRNA pairs conserved alongside the SCC progression model. Conserved enriched microRNA–mRNA pairs were visualized using the Cytoscape software ( http://www.cytoscape.org/ ). Quantitative real-time PCR validation analysis Separate cohorts of matched samples from patients consisting of NS, AK and cuSCC were processed as above. Commercially available Taqman (Life Technologies) probes were acquired for human miR-21 (000397), miR-31 (002279), PTPN14 (Hs00193643_m1), FAM134B (Hs00375273_m1), HMG2A (Hs00171569_m1), TIMP3 (Hs00165949_m1) and ARHGAP24 (Hs01097580_m1) and used in qRT-PCR based quantitation of expression in these tissues, as benchmarked to RNU6B (001093, microRNA) and 18S rRNA (Hs99999901, mRNA). Gene set enrichment analysis for TCGA tumour signatures GSEA was carried out using the GSEA software package [79] ( http://software.broadinstitute.org/gsea/index.jsp ) to assess the degree of similarity among the studied gene signatures. For each of the human or the mouse SCC progression transcriptome response, all genes were ranked by the fold change alongside the SCC progression model. To assess the relative association with multiple tumour progression signatures, we downloaded from the Cancer Genome Atlas (TCGA) ( https://tcga-data.nci.nih.gov/tcga/ ) gene expression data for 19 cancer cohorts, performed quantile normalization using the R statistical analysis system, and then inferred tumour progression transcriptome signature by imposing a fold change exceeding 2 ( P <0.05). We utilized separately the downregulated genes and the upregulated genes. Normalized Enrichment Score (NES) and adjusted q -values ( q <0.25) were computed utilizing the GSEA method, based on 1,000 random permutations of the ranked genes. We visualized combined NES scores for all the TCGA tumour development gene signatures and for our human and mouse SCC progression signatures using the Circos software [80] ( http://circos.ca/ ). Survival analysis for TCGA HNSCC with TP53 mutations We evaluated the survival prognostic power of cuSCC progression-associated gene signature using human specimen cohorts from the Cancer Genome Atlas (TCGA) ( https://tcga-data.nci.nih.gov/tcga/ ), specifically HNSCC which are TP53 -mutant. We first replaced the gene expression of each gene with the z -score within the cohort, then we computed the sum of z -scores for each sample by adding the z -score for upregulated genes and subtracting the z -score from downregulated genes. Specimens were sorted according to the sum z -score of the respective SCC progression gene signature; association with survival ( P <0.05, log-rank test) was evaluated by using the package Survival in the R statistical system ( https://cran.r-project.org/web/packages/survival/index.html ). Data availability Raw RNA and small RNA sequencing data from all human and mouse samples that were used to support the findings of this study have been deposited in NCBI/GEO with SuperSeries accession code GSE84194. The exome sequencing data that support the findings of this paper may be made available upon request from the corresponding author (K.Y.T.). These exome data are not publicly available due to them containing information that could compromise research participant privacy/consent. The data used to support the pan-cancer GSEA tumour signature analysis used publicly available Cancer Genome Atlas (TCGA) gene expression data, which can be accessed through the websites: ( https://tcga-data.nci.nih.gov/tcga/ ) ( https://gdc-portal.nci.nih.gov/ ). How to cite this article: Chitsazzadeh, V. et al . Cross-species identification of genomic drivers of squamous cell carcinoma development across preneoplastic intermediates. Nat. Commun. 7:12601 doi: 10.1038/ncomms12601 (2016).